Nonlinear spin-current enhancement enabled by spin-damping tuning When a magnon, the quanta of a spin excitation, is created in a magnet, this quasiparticle can split into two magnons, which triggers an angular momentum flow from the lattice to the spin subsystem. Although this process is known to enhance spin-current emission at metal/magnetic insulator interfaces, the role of interacting magnons in spintronic devices is still not well-understood. Here, we show that the enhanced spin-current emission is enabled by spin-damping tuning triggered by the redistribution of magnons. This is evidenced by time-resolved measurements of magnon lifetimes using the inverse spin Hall effect. Furthermore, we demonstrate nonlinear enhancement of the spin conversion triggered by scattering processes that conserve the number of magnons, illustrating the crucial role of spin-damping tuning in the nonlinear spin-current emission. These findings provide a crucial piece of information for the development of nonlinear spin-based devices, promising important advances in insulator spintronics. For more than half a century, the physics of spin dynamics has provided insight into the fundamental aspects of magnetism [1] , [2] , [3] , [4] . The collective excitations of localized spins coupled by the magnetic dipole and quantum exchange interactions are called spin waves or, in quantized form, magnons [5] . These quasiparticles, associated with the elementary magnetic excitation, are responsible for a flow of spin angular momentum, a spin current, in magnetic insulators, which are electrically inactive due to the frozen charge degrees of freedom, but magnetically active as a result of the interacting localized spins. In contrast to spin currents carried by conduction electrons in metals and semiconductors, which disappear within very short distances, spin currents in magnetic insulators persist over macroscopic distances owing to the substantially long lifetimes of the magnons relative to that of the conduction electron spins. The recent discovery of spin-carrier conversion from magnons to conduction electrons through dynamical spin exchange coupling at metal/magnetic insulator interfaces sheds new light on the physics of nonlinear spin dynamics, leading to the combination of spintronics with interacting magnons. In a metal/magnetic insulator junction, the excitation of nonequilibrium magnons in the magnetic layer emits a spin current into the attached metal through spin pumping [6] , [7] , [8] , [9] , [10] , [11] , [12] , [13] , [14] , [15] , [16] . The spin-current emission has been found to be enhanced through nonlinear magnon interactions [13] , [17] . Although the physics behind the spin-current enhancement is still not clear, this illustrates the crucial role of nonlinear spin dynamics and interacting magnons in spintronic devices. In this work, we demonstrate that the stabilized enhancement of the spin-current emission is enabled by spin-damping tuning, resulting from the redistribution of magnons due to the nonlinear magnon interactions. Of particular interest is the nonlinear three-magnon splitting, the splitting of one magnon into a pair of magnons (see Fig. 1a ). Since each magnon carries spin angular momentum, ℏ in the exchange limit, it is natural to expect that the splitting directly enhances the spin-current emission. However, this picture is valid only for the time scale of the spin-lattice relaxation; the steady-state enhancement of the spin-current emission is governed by the spin damping. Our direct measurements of the spin damping demonstrate that the stabilized enhancement of the spin-current emission is enabled by the long lifetime of the dipole-exchange secondary magnons created at the inflection point of the dispersion curve, where the negative dipolar dispersion is compensated by the positive exchange dispersion. We demonstrate, furthermore, that the spin-current emission can be enhanced even in the absence of the magnon splitting; we found enhanced spin-current emission triggered by scattering processes that conserve the number of magnons. These findings demonstrate the crucial role of magnon lifetimes in spintronic devices, opening a way for controlling nonlinear spin-current emission through spin-damping tuning. 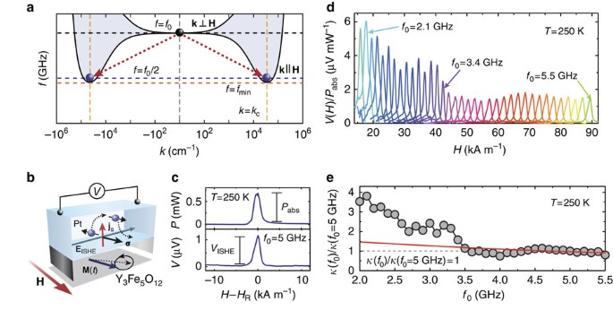Figure 1: Enhancement of spin-current emission induced by magnon splitting. (a) The magnon dispersion in YIG with a schematic of the three-magnon splitting, wherefandkare the frequency and wavenumber of magnons, respectively. The upper and lower boundaries of the magnon manifold correspond to the magnons propagating perpendicular and parallel to the applied field, respectively. The lowest frequency isf=fminatk=kc. (b) A schematic illustration of the Pt/YIG film.His the external static magnetic field andMis the magnetization.EISHEis the electric field generated by the ISHE from a spin current with the flow directionjsand spin polarization directionσ. (c) Magnetic field (H) dependence of the microwave absorptionPand electric voltageVfor the Pt/YIG film, where the microwave frequency and power aref0=5 GHz and 5 mW, respectively, atT=250 K.HRis the resonance field.PabsandVISHEare the definition of the magnitude of the microwave absorption and electric voltage, respectively. (d)V(H)/Pabsspectra for the Pt/YIG film atT=250 K for (from left to right)f0=2.0 GHz to 5.5 GHz with the step of 0.1 GHz. The curves in light blue, purple and light green indicated by the arrows are the experimental data forf0=2.1 GHz, 3.4 GHz and 5.5 GHz, respectively. (e)f0dependence of the ratioκ(f0,T)=VISHE(f0,T)/Pabs(f0,T), which characterizes the conversion efficiency of the angular momentum absorbed from microwaves into spin currents, atT=250 K. The solid line in red is the result of calculations based on the linear spin pumping theory. Figure 1: Enhancement of spin-current emission induced by magnon splitting. ( a ) The magnon dispersion in YIG with a schematic of the three-magnon splitting, where f and k are the frequency and wavenumber of magnons, respectively. The upper and lower boundaries of the magnon manifold correspond to the magnons propagating perpendicular and parallel to the applied field, respectively. The lowest frequency is f = f min at k = k c . ( b ) A schematic illustration of the Pt/YIG film. H is the external static magnetic field and M is the magnetization. E ISHE is the electric field generated by the ISHE from a spin current with the flow direction j s and spin polarization direction σ . ( c ) Magnetic field ( H ) dependence of the microwave absorption P and electric voltage V for the Pt/YIG film, where the microwave frequency and power are f 0 =5 GHz and 5 mW, respectively, at T =250 K. H R is the resonance field. P abs and V ISHE are the definition of the magnitude of the microwave absorption and electric voltage, respectively. ( d ) V ( H )/ P abs spectra for the Pt/YIG film at T =250 K for (from left to right) f 0 =2.0 GHz to 5.5 GHz with the step of 0.1 GHz. The curves in light blue, purple and light green indicated by the arrows are the experimental data for f 0 =2.1 GHz, 3.4 GHz and 5.5 GHz, respectively. ( e ) f 0 dependence of the ratio κ ( f 0 , T )= V ISHE ( f 0 , T )/ P abs ( f 0 , T ), which characterizes the conversion efficiency of the angular momentum absorbed from microwaves into spin currents, at T =250 K. The solid line in red is the result of calculations based on the linear spin pumping theory. Full size image Enhancement of spin-current emission The nonlinear spin-current emission from a magnetic insulator is investigated by measuring the voltage generated through the inverse spin Hall effect (ISHE) in a Pt/Y 3 Fe 5 O 12 (Pt/YIG) film, shown in Fig. 1b (details are outlined in Methods). Figure 1c shows the in-plane magnetic field, H , dependence of the microwave absorption intensity, P , measured by applying a 5 mW microwave with a fixed frequency of f 0 =5 GHz at T =250 K. Figure 1c shows that at H = H R =81.3 kA m −1 , H fulfills the ferromagnetic resonance condition: , where γ is the gyromagnetic ratio and M s is the saturation magnetization of the YIG layer. Around H = H R , we found voltage difference, V , between the ends of the Pt layer as shown in Fig. 1c . This provides evidence of spin-current emission from the YIG layer into the Pt layer; nonequilibrium magnons, excited by the magnetic resonance, emit a spin current into the Pt layer [18] , [19] , which is converted into an electric voltage by the ISHE in the Pt layer (see Fig. 1b ) [20] , [21] , [22] . The amplitude of the spin-current emission critically depends on the microwave excitation frequency, f 0 , because of the nonlinear dynamics of the interacting spins in the YIG layer. Figure 1d shows the field dependence of V ( H )/ P abs , measured at T =250 K for various f 0 values, where P abs is the microwave absorption intensity (see Fig. 1c ). Here V ( H )/ P abs characterizes the conversion efficiency of the angular momentum created by the microwave field into the spin current carried by the conduction electrons in the Pt layer. Notably, V ( H )/ P abs abruptly increases below f 0 = f c =3.4 GHz, while it is nearly constant for f 0 >3.5 GHz. To study the f 0 dependence of V ( H )/ P abs in detail, we plot κ ( f 0 , T )≡ V ISHE ( f 0 , T )/ P abs ( f 0 , T ) at different f 0 values in Fig. 1e , where V ISHE is the magnitude of the electric voltage. Figure 1e shows that κ ( f 0 , T =250 K) for f 0 >3.5 GHz is well-reproduced with a calculation based on the linear spin pumping model [23] (see the red line in Fig. 1e ), demonstrating that the enhancement of κ ( f 0 , T =250 K) at low f 0 originates from the nonlinearity of the spin dynamics in the YIG layer: the three-magnon splitting [17] . Here the microwave excitation power P in =5 mW is about 3 orders of magnitude larger than the threshold power of the three-magnon splitting [5] , [17] . Spin-current emission at various temperatures Importantly, the conversion efficiency κ is enhanced at low temperatures. 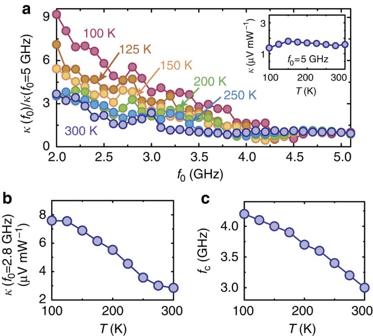Figure 2: Temperature dependence of spin-current enhancement. (a) Microwave excitation frequencyf0dependence ofκ(f0,T)=VISHE(f0,T)/Pabs(f0,T) for the Pt/YIG film at different temperatures. The inset shows temperatureTdependence ofκ(f0,T) in the linear regime:κ(f0=5 GHz,T), which is almost constant with temperature. (b) TemperatureTdependence of the spin-current enhancement factorκ(f0=2.8 GHz,T) at 2.8 GHz. The conversion efficiency increases with decreasing temperature. (c) TemperatureTdependence of the cut-off frequenciesfc, below which the three-magnon splitting becomes allowed.fcincreases with decreasing temperature due to the change of the magnon dispersion. Figure 2a shows the f 0 dependence of the conversion efficiency κ ( f 0 , T )= V ISHE ( f 0 , T )/ P abs ( f 0 , T ) at different temperatures T , where κ ( f 0 , T ) is divided by κ ( f 0 =5 GHz, T ) to omit the temperature dependent parameters relevant to the conversion efficiency from the spin current to the electric voltage such as the spin Hall angle, electrical conductivity and spin diffusion length in the Pt layer (see the inset to Fig. 2a ). Notably, κ ( f 0 , T ) clearly increases with decreasing temperature under the three-magnon splitting (see also Fig. 2b ). Figure 2a also shows that the cut-off frequency, f c , below which κ ( f 0 , T ) increases abruptly, increases with decreasing temperature (see Fig. 2c ). Figure 2: Temperature dependence of spin-current enhancement. ( a ) Microwave excitation frequency f 0 dependence of κ ( f 0 , T )= V ISHE ( f 0 , T )/ P abs ( f 0 , T ) for the Pt/YIG film at different temperatures. The inset shows temperature T dependence of κ ( f 0 , T ) in the linear regime: κ ( f 0 =5 GHz, T ), which is almost constant with temperature. ( b ) Temperature T dependence of the spin-current enhancement factor κ ( f 0 =2.8 GHz, T ) at 2.8 GHz. The conversion efficiency increases with decreasing temperature. ( c ) Temperature T dependence of the cut-off frequencies f c , below which the three-magnon splitting becomes allowed. f c increases with decreasing temperature due to the change of the magnon dispersion. Full size image We first discuss the T dependence of f c , which further supports that the three-magnon splitting is responsible for the enhancement of the spin-current emission increased at low temperatures. The three-magnon splitting creates a pair of magnons with opposite wavevectors and frequency f 0 /2 from the uniform magnon with a frequency of f 0 (see Fig. 1a ), following the energy and momentum conservation laws. Thus, the splitting process is only allowed for f 0 /2> f min , where f min is the minimum frequency of the magnon dispersion as shown in Fig. 1a . f min for the thin YIG film used in the present study can be obtained from the dipole-exchange magnon dispersion. The lowest branch of the magnon dispersion is expressed as [24] where Ω= ω H + ω M ( D / μ 0 M s ) K 2 , ω H = γμ 0 H , ω M = γμ 0 M s , K 2 = λ 2 + k 2 =(π/ L ) 2 + k 2 , and Q =( k / K ) 2 [1+( λ / K ) 2 (2/ kL ) [1+exp(− kL )]]. D is the exchange interaction constant, L is the thickness of the YIG layer and k is the wavenumber of the magnons. To obtain the exact condition f 0 /2> f min for the Pt/YIG film, a detailed calculation using equation (1) is necessary as discussed below. Before discussing in detail the condition for the three-magnon splitting based on the exact magnon dispersion, we first neglect the surface dipolar interactions in equation (1) for simplicity. f min under this approximation can be obtained in the limit of L →∞ as f min ≈ γμ 0 H . This relation with the resonance frequency shows that the condition f 0 /2> f min for the three-magnon splitting is satisfied when f 0 <(2/3) γμ 0 M s . This predicts that f c increases with M s due to the change in the magnon dispersion. We estimated M s of the Pt/YIG film from the resonance field H R using the Kittel formula (see Fig. 3a ) as shown in Fig. 3b . Using this result, we plot the relationship between f c and M s in Fig. 3c , which is consistent with the above discussion— f c increases with M s . Thus, the observed change in f c can be attributed to the change in the magnon dispersion, caused by the temperature variation of M s in the Pt/YIG film. 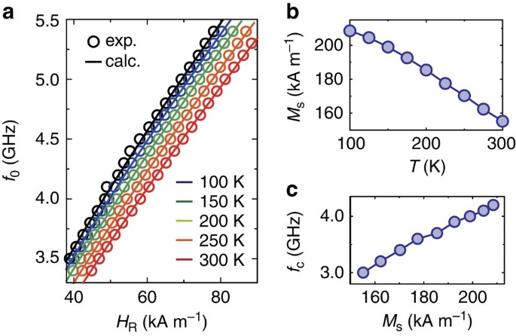Figure 3: Cut-off frequency and saturation magnetization. (a) Microwave excitation frequencyf0and the resonance fieldHRmeasured at different temperatures. The open circles are the experimental data and the solid curves are the fitting results using the Kittel formula. The resonance fieldHRdecreases with decreasing temperatureT. (b) TemperatureTdependence of the saturation magnetizationMs. The saturation magnetizationMsincreases with decreasing temperatureT. (c) The relationship between the cut-off frequencyfcand saturation magnetizationMs.fcincreases withMs, consistent with the prediction of the dipole-exchange magnon dispersion. Figure 3: Cut-off frequency and saturation magnetization. ( a ) Microwave excitation frequency f 0 and the resonance field H R measured at different temperatures. The open circles are the experimental data and the solid curves are the fitting results using the Kittel formula. The resonance field H R decreases with decreasing temperature T . ( b ) Temperature T dependence of the saturation magnetization M s . The saturation magnetization M s increases with decreasing temperature T . ( c ) The relationship between the cut-off frequency f c and saturation magnetization M s . f c increases with M s , consistent with the prediction of the dipole-exchange magnon dispersion. Full size image The experimentally measured temperature dependences of f c and M s shown in Figs 2c and 3b illustrate the exact magnon dispersion of the Pt/YIG film at each temperature using equation (1). When the external magnetic field H is varied, the magnon dispersion is shifted in frequency space and the relationship between the frequencies f 0 /2 and f min also changes. 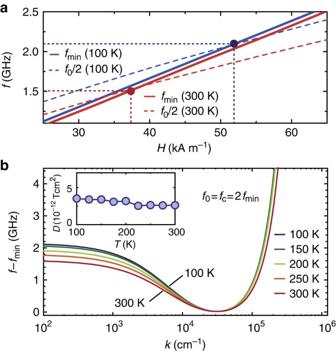Figure 4: Magnon dispersions. (a) Magnetic field (H) dependence of the frequencyf0/2 and those of the frequencyfminforT=100 and 300 K (seeFig. 1a). The points of interception determine the onset of the region where the three-magnon splitting is allowed. (b) The lowest-energy branch of the magnon spectra for the Pt/YIG film calculated forf0=fc=2fmin, where the three-magnon splitting is allowed. The dispersions were calculated forH=37.0 kA m−1, 42.3 kA m−1, 45.8 kA m−1, 49.5 kA m−1and 52.0 kA m−1atT=300 K, 250 K, 200 K, 150 K and 100 K, respectively.fminis the lowest frequency in the dispersions. The inset showsTdependence of the exchange interaction constantDestimated from theTdependence offc. Figure 4a shows a plot of the H dependences of f 0 /2 and f min at T =100 and 300 K, where f 0 /2 was calculated using the Kittel formula with the experimentally obtained M s . f min was plotted by finding the minimum frequency of the magnon dispersion using equation(1). The crossing points of f 0 /2 and f min correspond to the cut-off frequency f c , where f min and the crossing point can be varied by changing the exchange interaction constant D ; D for which the crossing point reproduces the measured f c value at different temperatures is plotted in the inset to Fig. 4b . The experimentally obtained D is almost temperature independent, consistent with the literature [25] . Using the values of M s and D , we plot the lowest branch of the magnon dispersion at the cut-off frequency, f 0 = f c =2 f min , for different temperatures in Fig. 4b . Figure 4b shows that the shape of the lowest branch of the magnon dispersion changes slightly by changing temperature, which is the origin of the temperature dependence of the cut-off frequency. Figure 4: Magnon dispersions. ( a ) Magnetic field ( H ) dependence of the frequency f 0 /2 and those of the frequency f min for T =100 and 300 K (see Fig. 1a ). The points of interception determine the onset of the region where the three-magnon splitting is allowed. ( b ) The lowest-energy branch of the magnon spectra for the Pt/YIG film calculated for f 0 = f c =2 f min , where the three-magnon splitting is allowed. The dispersions were calculated for H =37.0 kA m −1 , 42.3 kA m −1 , 45.8 kA m −1 , 49.5 kA m −1 and 52.0 kA m −1 at T =300 K, 250 K, 200 K, 150 K and 100 K, respectively. f min is the lowest frequency in the dispersions. The inset shows T dependence of the exchange interaction constant D estimated from the T dependence of f c . Full size image The observed enhancement of the spin-current emission is enabled by spin-damping tuning triggered by the redistribution of magnons due to the nonlinear magnon scattering. Here note that the steady-state spin-current emission from the magnetic insulator is stabilized by balancing the creation and decay of the magnons; the steady-state angular momentum stored in the spin system is governed by the magnon damping. Assuming that the spin current emitted from the magnetic insulator is proportional to the total number of nonequilibrium magnons [26] , [27] , and using the energy balance relation P abs =∑ k ℏ ω k η k N k , we find that the conversion efficiency κ = V ISHE / P abs is proportional to the spin-lattice relaxation time τ of the pumped system: κ ∝ τ . The relaxation rate 1/ τ is given by where N k and η k are the number and the damping of nonequilibrium magnons with the wavenumber k , respectively, and N t =∑ k N k is the total number of nonequilibrium magnons in the system. This simple model provides a general picture of the nonlinear spin-current emission in the presence of magnon scatterings; the above model indicates that the spin-current emission can be enhanced through the magnon redistribution in a system with η 0 > η q , where η 0 and η q are the damping of the uniform and secondary magnons, respectively. In this system, the magnon redistribution triggered by magnon interactions destroys the magnons with the large-damping η 0 and creates the magnons with the small-damping η q , changing the relative weight N k / N t in equation (2) and decreasing the dissipation rate 1/ τ of the angular momentum from the spin system to the lattice. This spin-damping tuning, triggered by the magnon redistribution, increases the steady-state angular momentum stored in the spin system, giving rise to the stabilized enhancement of the spin-current emission. The spin damping 1/ τ can be measured directly by monitoring the temporal evolution of the spin-current emission using the ISHE, which provides direct evidence that the spin damping plays a key role in the spin-current enhancement. 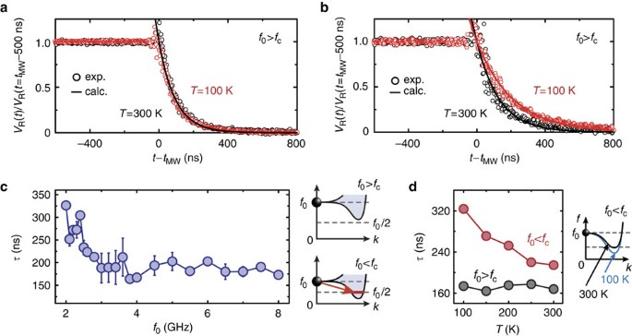Figure 5: Magnon lifetimes. (a) Electric voltage due to the ISHE,VR(t), at the resonance fieldH=HRas a function of timetatT=100 K (the red circles) and 300 K (the black circles) forf0=8 GHz>fc. Att=tMW, the microwaves were switched off. (b)VR(t) forf0=2.8 GHz<fcatT=100 K (the red circles) and 300 K (the black circles). (c) Microwave excitation frequencyf0dependence of the decay timeτof theVR(t) signal. The magnon dispersion are also shown forf0>fcandf0<fc. The dotted lines showf0andf0/2. The red arrow indicates the magnon splitting. (d)Tdependence of the decay timeτof theVR(t) signal forf0=8.0 GHz (the black circles) andf0=2.8 GHz (the red circles). A schematic illustration of the lowest branch of the magnon dispersion under the splitting condition (f0<fc) forT=100 K (the blue curve) and 300 K (the black curve) at the same excitation frequency is also shown. Figure 5a shows the temporal evolution of the electric voltage due to the ISHE in the absence of the three-magnon splitting: f 0 =8 GHz> f c . The temporal profile of the ISHE voltage, V R ( t ), at the resonance field, H = H R , was measured by applying a microwave pulse that was switched off at t = t MW . Figure 5a shows that V R ( t ) decays exponentially after switching off the microwaves; the spin-current emission decreases with time due to the dissipation of the angular momentum from the spin system to the lattice in the YIG layer [28] . The spin-current decay was also observed at f 0 =2.8 GHz< f c as shown in Fig. 5b , where the dipole-exchange magnons are created by the three-magnon splitting. For these results, we extracted the relaxation time, τ , by fitting the voltage with V R ( t )/ V R ( t = t MW −500 ns)=exp(−2 t / τ ) for t > t MW . The extracted relaxation time τ for different f 0 at T =300 K is shown in Fig. 5c . Figure 5c shows that τ is almost constant for f 0 > f c . In contrast, τ increases with decreasing the excitation frequency for f 0 < f c , reminiscent of the f 0 dependence of κ shown in Fig. 2a . These results, therefore, demonstrate the direct relationship between the spin damping and the conversion efficiency in the nonlinear spin-current emission. Figure 5: Magnon lifetimes. ( a ) Electric voltage due to the ISHE, V R ( t ), at the resonance field H = H R as a function of time t at T =100 K (the red circles) and 300 K (the black circles) for f 0 =8 GHz> f c . At t = t MW , the microwaves were switched off. ( b ) V R ( t ) for f 0 =2.8 GHz< f c at T =100 K (the red circles) and 300 K (the black circles). ( c ) Microwave excitation frequency f 0 dependence of the decay time τ of the V R ( t ) signal. The magnon dispersion are also shown for f 0 > f c and f 0 < f c . The dotted lines show f 0 and f 0 /2. The red arrow indicates the magnon splitting. ( d ) T dependence of the decay time τ of the V R ( t ) signal for f 0 =8.0 GHz (the black circles) and f 0 =2.8 GHz (the red circles). A schematic illustration of the lowest branch of the magnon dispersion under the splitting condition ( f 0 < f c ) for T =100 K (the blue curve) and 300 K (the black curve) at the same excitation frequency is also shown. Full size image The observed spin-current enhancement and spin-damping tuning is realized by the small damping and long-lived nature of the dipole-exchange secondary magnons created by the three-magnon splitting. When f 0 < f c , the three-magnon splitting creates the dipole-exchange secondary magnons with wavevectors of k =± q from the k = 0 uniform magnons near the bottom of the magnon dispersion as shown in Fig. 1a . Although the damping of the uniform magnon is dominated by the elastic two-magnon scattering due to nonuniformities, where a magnon is destroyed and another magnon at the same frequency is created [29] , the two-magnon scattering can be suppressed for the dipole-exchange secondary magnons created by the three-magnon splitting. For the secondary magnons, because of the nearly zero group velocity due to the competition of the magnetic dipole and quantum exchange interactions, the scattering events due to nonuniformities are suppressed, resulting in the long lifetime, or the small damping. In the presence of the three-magnon splitting, the dynamics of these uniform and secondary magnons are modelled as and , because short wavelength magnons do not couple to the microwave field. n k ( k =0, ± q ) is the number of the magnons with the wavenumber k and the damping η k . is the thermodynamic equilibrium value of n k . P abs is the absorbed microwave power and ω 0 =2π f 0 . Here for simplicity, we assume that the damping due to the three-magnon splitting as η 3s =Γ 3s ( n q + n − q ), where Γ 3s is the splitting strength. [5] , [30] Notably, the splitting strength Γ 3s increases with the decreasing excitation frequency f 0 , because the number of the degenerate states at f 0 /2 available for the splitting increases by decreasing f 0 (see also the schematic illustrations in Fig. 5c ) [30] . Thus, by decreasing f 0 below the cut-off frequency, the relative number of the small-damping dipole-exchange secondary magnons increases and that of the large-damping uniform magnons decreases (see also equation (2)), resulting in the long lifetime τ of the spin system as demonstrated in Fig. 5c . The effect of the creation of an additional magnon through the splitting on κ becomes evident in a strong excitation condition. For Γ 3s ≠0, from the above rate equations, the number of the nonequilibrium uniform magnons can be expressed as , where n q ,− q ≡ n q = n − q and η q ,− q ≡ η q = η − q . In the limit of strong excitation, that is, , the number of the nonequilibrium uniform magnons is limited to N 0 ≃ η q ,− q /2Γ 3s . Thus, in this condition, and N t ≃ 2 N q ,− q , resulting in κ 3s = V ISHE / P abs ∝ 2/ η q ,− q because of the approximated energy balance relation . The factor 2 arises from the fact that the three-magnon splitting creates two magnons from one magnon. Although the three-magnon splitting triggers the angular momentum flow from the lattice, the creation of the secondary magnons also affects the inherent dissipation of the angular momentum from the magnons to the lattice; when the redistribution of magnons creates secondary magnons with exceptionally short lifetimes, this redistribution process enhances the inherent dissipation of the angular momentum of the spin system or decreases τ of the system, masking the angular momentum flow from the lattice triggered by the nonlinear magnon interaction. Thus, in the steady state, it is nontrivial whether the magnon splitting increases or decreases the nonequilibrium angular momentum stored in the spin system. Since in the absence of the splitting, Γ 3s =0, the conversion efficiency is expressed as κ linear ∝ 1/ η 0 , the spin-current emission can be enhanced by the three-magnon splitting when the damping of the uniform and secondary magnons satisfies κ 3s / κ linear =2 η 0 / η q ,− q >1; the creation of long-lived magnons with a damping of η q ,− q (<2 η 0 ) through the nonlinear magnon scattering is responsible for the enhancement of the spin-current emission. The temperature dependence of the conversion efficiency κ shown in Fig. 2b further demonstrates that the spin-current emission is governed by the spin damping of the system. Figure 5a shows that the decay time of V R ( t ) is almost independent of temperature when f 0 =8 GHz> f c , that is, in the absence of the three-magnon splitting. In contrast, the voltage decay time varies by changing the temperature at f 0 =2.8 GHz< f c , as shown in Fig. 5b . The temperature dependence of the decay time, τ , is summarized in Fig. 5d . This result shows that the magnon relaxation time τ increases with decreasing temperature under the three-magnon splitting, consistent with the experimentally obtained temperature dependence of κ shown in Fig. 2b . At the fixed excitation frequency f 0 , the number of the available states at f 0 /2 for the splitting increases with decreasing temperature (see Fig. 5d ). This indicates that the relative number of the small-damping secondary magnons increases with decreasing temperature, which reduces the damping of the spin system through the splitting. The damping of the secondary magnon itself is also expected to be reduced with decreasing temperature, since the damping of the dipole-exchange magnon is dominated by the three-particle processes, which is almost proportional to temperature [29] , [31] . Therefore, by decreasing temperature, both the splitting strength and the damping of the secondary magnons tend to increase the relaxation time of the spin system, giving rise to the experimentally observed longer τ at low temperatures. The direct measurements of the spin damping at different frequencies and temperatures shown in Fig. 5 provide evidence that the creation of the long-lived secondary dipole-exchange magnons through the redistribution is essential for the enhancement of the spin-current emission. This picture is further evidenced by microwave excitation power P in dependence of the conversion efficiency κ ( P in )= V ISHE ( P in )/ P abs ( P in ) for the Pt/YIG film shown in Fig. 6a . The applied microwave excitation frequency was f 0 =7.6 GHz> f c , that is, the three-magnon splitting is prohibited in this measurement. For P in < P th , the conversion efficiency is constant, consistent with the spin-current emission in the linear regime [32] ; the emitted spin current is proportional to P in . However, κ ( P in ) clearly increases by increasing P in for P in > P th , demonstrating the enhancement of the spin conversion efficiency without the splitting of a pumped magnon, or without breaking the angular momentum conservation of the spin subsystem. Notably, κ ( P in ) shows a clear threshold power P th , indicating that the four-magnon scattering [33] , [34] , where two magnons are created with the annihilation of two other magnons, is responsible for the enhanced spin-current emission. 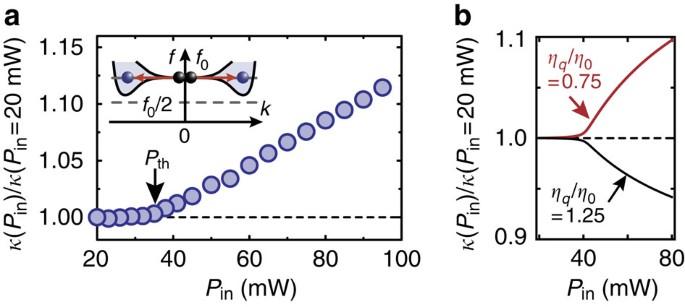Figure 6: Nonlinear spin-current emission. (a), Microwave excitation powerPindependence ofκ(Pin)≡VISHE(Pin)/Pabs(Pin) for the Pt/YIG film measured at room temperature. The applied microwave excitation frequency wasf0=7.6 GHz>fc, that is, the three-magnon splitting is prohibited. The black arrow indicates the threshold powerPth. ForPin<Pth, the conversion efficiency is constant, consistent with the spin-current emission in the linear regime. However,κ(Pin) clearly increases by increasingPinforPin>Pth, demonstrating the enhancement of the spin conversion efficiency without the splitting of a pumped magnon. (b) CalculatedPindependence ofκ(Pin) using equation (3) forηq/η0=0.75 (the red curve) andηq/η0=1.25 (the black curve), whereη0andηqare the damping of the uniform and secondary magnons, respectively.Pth=40 mW andηsp=0.005γwere used for the calculations. Whenηq/η0=0.75, the conversion efficiencyκ(Pin) increases withPinforPin>Pththrough the creation of the small-damping secondary magnons. Figure 6: Nonlinear spin-current emission. ( a ), Microwave excitation power P in dependence of κ ( P in )≡ V ISHE ( P in )/ P abs ( P in ) for the Pt/YIG film measured at room temperature. The applied microwave excitation frequency was f 0 =7.6 GHz> f c , that is, the three-magnon splitting is prohibited. The black arrow indicates the threshold power P th . For P in < P th , the conversion efficiency is constant, consistent with the spin-current emission in the linear regime. However, κ ( P in ) clearly increases by increasing P in for P in > P th , demonstrating the enhancement of the spin conversion efficiency without the splitting of a pumped magnon. ( b ) Calculated P in dependence of κ ( P in ) using equation (3) for η q / η 0 =0.75 (the red curve) and η q / η 0 =1.25 (the black curve), where η 0 and η q are the damping of the uniform and secondary magnons, respectively. P th =40 mW and η sp =0.005 γ were used for the calculations. When η q / η 0 =0.75, the conversion efficiency κ ( P in ) increases with P in for P in > P th through the creation of the small-damping secondary magnons. Full size image The enhanced spin-current emission induced by the scattering process that conserve the number of magnons, that is, the four-magnon scattering, demonstrates the general picture of the role of the magnon interactions in the nonlinear spin-current emission: the spin-damping tuning triggered by the magnon redistribution. In the absence of the redistribution of magnons, the angular momentum relaxation rate from the spin system to the lattice is 1/ τ ≃ η 0 because of N t ≃ N 0 . Although the four-magnon scattering creates dipole-exchange magnons at the excitation frequency f 0 not at f 0 /2, the lifetime of these magnons can be longer than that of the uniform magnon because of the small group velocity [35] . Thus, even in the absence of the three-magnon splitting, the four-magnon scattering can decrease the relaxation rate of the spin system, 1/ τ , through the annihilation of the uniform magnons with large η 0 and creation of dipole-exchange magnons with small η q , resulting in the steady-state enhancement of the angular momentum stored in the spin system or the enhanced spin-current emission shown in Fig. 6a . This is further supported by a rate equation approach for the four-magnon scattering [33] , [36] , [37] : d N 0 /d t =−[ η 0 + η sp f ( P in )] N 0 + P abs / ℏ ω 0 and d( N t − N 0 )/d t =− η q ( N t − N 0 )+ η sp f ( P in ) N 0 , where . η sp is the decay constant of the uniform precession to degenerate magnons at f 0 due to scattering from sample inhomogeneities. To keep the discussion simple, we define η q as the average decay rate to the thermodynamic equilibrium of the degenerate secondary magnons. P th is the threshold power for the four-magnon scattering and χ ″ is the imaginary part of the susceptibility. P abs = ω 0 χ ″ h 2 and h is the applied microwave field strength. The steady-state solution of the above rate equation gives where κ ( P in ) ∝ N t / P abs and χ ″=(2 γM s )/( η 0 + η sp f ( P in )). Figure 6b shows the conversion efficiency κ ( P in ) calculated using equation (3) for η q / η 0 =0.75 (the red curve) and η q / η 0 =1.25 (the black curve) with the assumption of V ISHE ∝ N t . In a system with η q / η 0 =1.25, κ ( P in ) decreases with P in for P in > P th , since the scattering process increases the relative number of the large-damping magnons and increases the dissipation rate of the angular momentum stored in the spin system (see equation (2)). In contrast, in a system with η q / η 0 =0.75, the four-magnon scattering increases the relative number of the small-damping magnons and decreases the damping of the spin system, resulting in the enhanced spin-current emission, which is consistent with the experimental observation shown in Fig. 6a . The observed enhancement of the spin-current emission demonstrates the crucial role of the spin damping affected by nonlinear magnon interactions in spintronic devices. The damping of the spin system can be directly quantified using the time-resolved measurement of the spin-current emission under various conditions, providing a way for further development of the physics of nonlinear spin conversion. These findings shed new light on nonlinear spin dynamics, promising important advances in spintronics with interacting magnons. Sample preparation The sample used in this study is a Pt/YIG film. A single-crystal YIG (111) film (3 × 5 mm 2 ) with a thickness of 5 μm was grown on a Gd 3 Ga 5 O 12 (111) substrate by liquid phase epitaxy. A 10-nm-thick Pt layer was sputtered in an Ar atmosphere on top of the film and two electrodes were attached to the edges of the Pt layer for voltage measurements. ISHE voltage and microwave absorption measurements The Pt/YIG film was placed at the centre of a coplanar waveguide, where a microwave signal with a frequency of f 0 was applied to the input of the signal line. The signal line of the coplanar waveguide is 500 μm wide and the gaps between the signal line and the ground lines are designed to match the characteristic impedance of 50 Ω. An in-plane external magnetic field was applied parallel to the signal line, such that the static magnetic field is perpendicular to the dynamic magnetic field produced by the microwave current. The microwave power absorbed by the sample P abs was measured by monitoring the transmitted output power. How to cite this article: Sakimura, H. et al. Nonlinear spin-current enhancement enabled by spin-damping tuning. Nat. Commun. 5:5730 doi: 10.1038/ncomms6730 (2014).